The Pan-Cancer analysis of pseudogene expression reveals biologically and clinically relevant tumour subtypes Although individual pseudogenes have been implicated in tumour biology, the biomedical significance and clinical relevance of pseudogene expression have not been assessed in a systematic way. Here we generate pseudogene expression profiles in 2,808 patient samples of seven cancer types from The Cancer Genome Atlas RNA-seq data using a newly developed computational pipeline. Supervised analysis reveals a significant number of pseudogenes differentially expressed among established tumour subtypes and pseudogene expression alone can accurately classify the major histological subtypes of endometrial cancer. Across cancer types, the tumour subtypes revealed by pseudogene expression show extensive and strong concordance with the subtypes defined by other molecular data. Strikingly, in kidney cancer, the pseudogene expression subtypes not only significantly correlate with patient survival, but also help stratify patients in combination with clinical variables. Our study highlights the potential of pseudogene expression analysis as a new paradigm for investigating cancer mechanisms and discovering prognostic biomarkers. Pseudogenes are dysfunctional copies of protein-coding genes that have lost their ability to encode amino acids through the accumulation of deleterious mutations such as in-frame stop codons and frame-shift insertions/deletions [1] . In the human genome, there are pseudogene copies for many protein-coding genes: for example, the ENCODE project recently annotated ~\n15,000 human pseudogenes [2] . Importantly, a large fraction of pseudogenes are transcriptionally active [2] . Despite their huge number and prevalent occurrence in the genome, pseudogenes have long been considered as nonfunctional and assumed to evolve neutrally [3] . In recent years, a growing body of evidence has strongly suggested that individual pseudogenes play critical roles in human diseases such as cancer [4] , [5] . For example, NANOG and OCT4 are essential transcription factors for the maintenance of pluripotency in embryonic stem cells [6] , [7] , while their pseudogenes, NANOGP1 and POU5F1P1, are aberrantly expressed in human cancers [8] . Poliseno et al. [9] showed that the pseudogenes of key cancer genes (for example, PTENP1 and KRASP1) can regulate the expression of their wild-type (WT) cognate genes by sequestering miRNAs. More recently, Kalyana-Sundaram et al. [10] performed the first genome-wide characterization of pseudogene expression in human cancers using the RNA-seq approach and revealed a considerable number of pseudogenes with a lineage- or cancer-specific expression pattern. These studies provide key insights into the potential role of transcribed pseudogenes in tumour biology. However, due to the limited number of patient samples surveyed in previous studies, the biomedical significance of pseudogene expression in cancer cannot be fully assessed. In particular, it remains unclear whether pseudogene expression can effectively characterize the tumour heterogeneity within a specific cancer type and represent a meaningful dimension for patient stratification. Therefore, it is essential to perform a systematic analysis across large patient sample cohorts to evaluate the potential clinical utility of pseudogene expression. Taking advantage of large-scale RNA-seq transcriptomic data recently made available from The Cancer Genome Atlas (TCGA) project, we developed a computational pipeline and characterized the pseudogene expression profiles of a large number of patient samples in a wide range of cancer types. With this unprecedented dataset, we first identified differentially expressed pseudogenes among established tumour subtypes and demonstrated the predictive power in classifying clinical tumour subtypes of endometrial cancer. Then we examined the biomedical relevance of the tumour subtypes revealed by pseudogene expression and assessed the potential clinical utility of pseudogene expression subtypes in terms of predicting patient survival. Taken together, our results indicate that expressed pseudogenes represent an exciting paradigm for investigating cancer-related molecular mechanisms and discovering effective prognostic biomarkers. Overview of pseudogene expression in multiple cancer types To comprehensively detect expressed pseudogenes and quantify their expression levels in human cancer, we developed a computational pipeline, as shown in Fig. 1 . First, we combined the latest pseudogene annotations from the Yale Pseudogene database [11] and the GENCODE Pseudogene Resource [2] and filtered those pseudogene exons overlapped with any known protein-coding genes. Second, to address the issue of potential cross-mapping between pseudogenes and their WT-coding genes, we evaluated the sequence uniqueness of each exon of a pseudogene [12] , and only retained those pseudogenes containing exon(s) with sufficient alignability for further characterization (Methods). Third, we filtered those reads mapped to multiple genomic locations from TCGA BAM files. 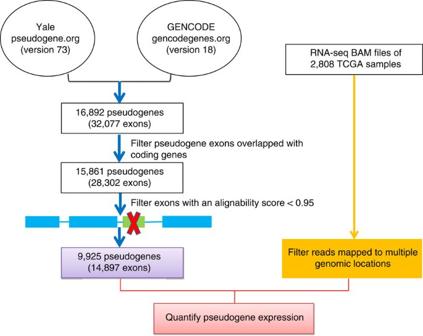Figure 1: A computational pipeline to quantify the expression of pseudogenes from TCGA RNA-seq data. First, we combined the latest pseudogene annotations from the Yale Pseudogene database and the GENCODE Pseudogene Resource, and filtered those pseudogene exons that overlapped with any known protein-coding genes. Second, we evaluated the sequence uniqueness of each exon of a pseudogene, and only retained those pseudogenes containing exon(s) with sufficient alignability for further characterization. Third, we filtered those reads mapped to multiple genomic locations from TCGA BAM files. Through analysing more than 378 billion RNA-seq reads, we measured the expression levels of 9,925 pseudogenes (based on the regions of high sequence uniqueness) in 2,808 samples of seven cancer types ( Table 1 ). These cancer types included breast invasive carcinoma (BRCA) [13] , glioblastoma multiforme (GBM) [14] , kidney renal clear cell carcinoma (KIRC) [15] , lung squamous cell carcinoma (LUSC) [16] , ovarian serous cystadenocarcinoma (OV) [17] , colorectal carcinoma (CRC) [18] and uterine corpus endometrioid carcinoma (UCEC) [19] . Figure 1: A computational pipeline to quantify the expression of pseudogenes from TCGA RNA-seq data. First, we combined the latest pseudogene annotations from the Yale Pseudogene database and the GENCODE Pseudogene Resource, and filtered those pseudogene exons that overlapped with any known protein-coding genes. Second, we evaluated the sequence uniqueness of each exon of a pseudogene, and only retained those pseudogenes containing exon(s) with sufficient alignability for further characterization. Third, we filtered those reads mapped to multiple genomic locations from TCGA BAM files. Full size image Table 1 Summary of The Cancer Genome Atlas RNA-seq data sets used in this study. Full size table Among the seven cancer types we surveyed, five data sets (BRCA, GBM, LUSC, KIRC and OV) had been obtained through a paired-end sequencing strategy, while the other two (CRC and UCEC) had resulted from a single-end sequencing strategy. Moreover, samples in the paired-end group had many more mappable reads than those in the single-end group ( Table 1 , Supplementary Fig. 1 ). For each cancer type, we observed generally weak correlations between the expression level of pseudogenes and WT genes, which is consistent with the previous study [10] ( Supplementary Fig. 2 ). In general, the expression correlation between a pseudogene and its WT-coding gene could be affected by three factors: (i) the sequence similarity between the pseudogene/gene pair; (ii) the molecular mechanisms through which the pseudogene functions; and (iii) the detection sensitivity given the setting of RNA-seq experiments. We detected more expressed pseudogenes (with an average reads per kilobase per million (RPKM)) [20] cutoff ≥0.3, as in the literature [21] , [22] ) in the paired-end group (OV: 670, KIRC 712, LUSC 813, BRCA: 747 and GBM, 875) than in the single-end group (UCEC, 181 and CRC, 168) ( Table 1 ). Both the larger numbers of sequenced reads and the higher read mapping accuracy in the paired-end group contributed to this difference. Indeed, the two groups showed distinct global patterns of pseudogene expression ( Supplementary Fig. 3 ). Considering the potential confounding factors (for example, sequencing strategy and read coverage) for quantifying the pseudogene expression, we performed the cross-tumour analyses for these two groups separately. As observed in [10] , we detected some tumour lineage-specific pseudogenes (296 from the paired-end group and 41 from the single-end group, Supplementary Fig. 4 ). In addition, for three cancer types with available RNA-seq data from nontumour tissue samples, we identified differentially expressed pseudogenes between tumour and nontumour samples (54 in BRCA, 110 in KIRC and 138 in LUSC, Supplementary Fig. 5 ). Supervised analysis of pseudogene expression on tumour subtypes However, the tumour lineage-specific or cancer-specific pseudogenes identified above may only reflect biological characteristics unique to distinct tissue types rather than key biological factors involved in tumorigenesis. Therefore, it is more critical and informative to examine the expression patterns of pseudogenes among tumour subtypes within a disease. For several cancer types with established tumour subtypes, we performed the supervised analysis and revealed substantial numbers of pseudogenes with significant differential expression: 48 in UCEC (endometrioid vs serous) [23] , 138 in LUSC (basal, classical, primitive and secretory) [16] , 71 in GBM (classical, mesenchymal, neural and proneural) [24] and 547 in BRCA (PAM50 subtypes: luminal A, luminal B, basal-like, Her2-enriched and normal-like) [25] (Methods, Fig. 2a , Supplementary Data 1 ). This analysis not only reveals a large number of pseudogenes with potential biomedical significance, but also provides new insights into known oncogenic pseudogenes. For example, ATP8A2P1 has been reported to play a growth regulatory role and to be expressed in a BRCA-specific manner [10] . Through the analysis of the large BRCA sample cohort, we further demonstrated that this pseudogene shows significant expression variation across subtypes, with the highest level in luminal A and the lowest level in the basal-like subtype (analysis of variance P <2.2 × 10 −16 , Fig. 2b ). 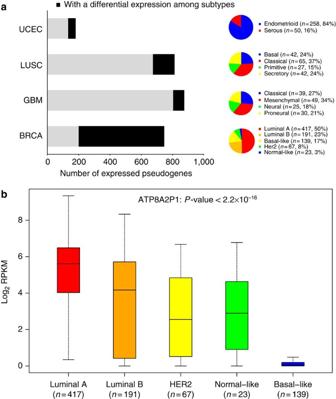Figure 2: Identification of differentially expressed pseudogenes among established tumour subtypes. (a) Numbers of significantly differentially expressed pseudogenes in multiple cancer types. For each cancer type, the whole bar represents the number of expressed pseudogenes (meanRPKM≥0.3) in the analysis; the black part represents the number of expressed pseudogenes with a detected significance for differential expression among tumour subtypes (t-test or single-factor analysis of variance, correctedP<0.05) and the pie chart shows the sample numbers and percentages in each cancer type. (b) The box plot for the expression pattern of ATP8A2P1 in 837 BRCA samples based on PAM50 subtypes: luminal A (n=417), luminal B (n=191), basal-like (n=139), Her2-enriched (n=67) and normal-like (n=23). The boxes show the median±1 quartile, with whiskers extending to the most extreme data point within 1.5 interquartile range from the box boundaries. Figure 2: Identification of differentially expressed pseudogenes among established tumour subtypes. ( a ) Numbers of significantly differentially expressed pseudogenes in multiple cancer types. For each cancer type, the whole bar represents the number of expressed pseudogenes (mean RPKM ≥0.3) in the analysis; the black part represents the number of expressed pseudogenes with a detected significance for differential expression among tumour subtypes ( t -test or single-factor analysis of variance, corrected P <0.05) and the pie chart shows the sample numbers and percentages in each cancer type. ( b ) The box plot for the expression pattern of ATP8A2P1 in 837 BRCA samples based on PAM50 subtypes: luminal A ( n =417), luminal B ( n =191), basal-like ( n =139), Her2-enriched ( n =67) and normal-like ( n =23). The boxes show the median±1 quartile, with whiskers extending to the most extreme data point within 1.5 interquartile range from the box boundaries. Full size image Among the tumour subtypes we surveyed, endometrioid and serous endometrial tumours are two major histological subtypes for UCEC, which are defined independently from the molecular data. Importantly, these two subtypes have distinct pathological characteristics and clinical behaviours. Early-stage endometrioid cancers are often treated with surgery only, whereas serous tumours are usually treated with chemotherapy [26] . Therefore, subtype classification is crucial for selecting appropriate therapy. To assess the clinical utility of pseudogene expression in UCEC, we applied a rigorous machine-learning approach to assess the power of expressed pseudogenes in classifying these two subtypes. First, we divided the TCGA UCEC samples into training and test sets according to their tissue source sites ( Fig. 3a ). Second, within the training set, we applied three well-established machine-learning algorithms (random forest (RF) [27] ; support vector machine (SVM) [28] ; and logistic regression (LR)) and evaluated their performance based on the area under the receiveroperating characteristics curve (area under curve (AUC) score) through fivefold cross-validation (Methods, Fig. 3b ). Strikingly, we found that the pseudogene expression profile can accurately classify these two histological subtypes (RF, AUC score=0.944, SVM, AUC score=0.962, LR, AUC score=0.892, Fig. 3c ). Moreover, the best-performing algorithm, SVM, achieved a high AUC of 0.922 on the independent test set ( Fig. 3d ). The predictive power of pseudogene expression is comparable with those achieved by the mRNA expression profiles, suggesting that both pseudogene and mRNA expression can classify the UCEC subtypes independently ( Supplementary Fig. 6 ). These results indicate that pseudogene expression can effectively capture clinically relevant information and may provide an independent approach to validate the classification of tumour subtypes. 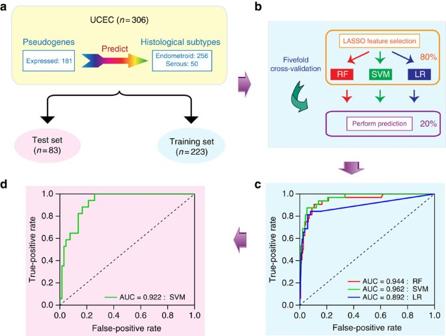Figure 3: The predictive power of pseudogene expression in classification of UCEC subtypes. (a) The UCEC dataset (n=306) was split into training (n=223) and test (n=83) sets. (b) Schematic representation of feature selection and classifiers building through fivefold cross-validation within the training set. (c) The receiver operating characertistic curves of the three classifiers based on the cross-validation within the training set. (d) The receiver operating characertistic curve from applying the best-performing classifier (SVM) built from the whole training set to the test set. Figure 3: The predictive power of pseudogene expression in classification of UCEC subtypes. ( a ) The UCEC dataset ( n =306) was split into training ( n =223) and test ( n =83) sets. ( b ) Schematic representation of feature selection and classifiers building through fivefold cross-validation within the training set. ( c ) The receiver operating characertistic curves of the three classifiers based on the cross-validation within the training set. ( d ) The receiver operating characertistic curve from applying the best-performing classifier (SVM) built from the whole training set to the test set. Full size image Assessment of pseudogene expression tumour subtypes Cancer is a complex disease involving multiple layers of aberrations that cannot be sufficiently captured by any single type of molecular data. In recent years, various ‘omic’ data, such as mRNA expression, microRNA expression, DNA methylation, somatic copy number alteration and protein expression, have been widely used to classify tumour samples into different molecular subtypes [13] , [14] , [15] , [16] , [17] , [18] , [19] . The integrative analysis across these molecular subtypes, especially through the efforts in TCGA, often provide crucial insights into pathobiology and help stratify patients for predicting prognosis and selecting effective treatment. To complement the supervised analysis in the above section, we next performed unsupervised analyses and explored the biomedical relevance of tumour subtypes based on pseudogene expression profiles. For each cancer type, we selected the pseudogenes with the most variable expression (500 for each cancer in the paired-end group and 100 for each cancer in the single-end group, respectively) and used non-negative matrix factorization (NMF) [29] to classify tumour samples into subtypes (clusters). Strikingly, in multiple cancer types, we observed that subtypes based on pseudogene expression had high concordance with other molecular subtypes ( Fig. 4a , χ 2 tests). 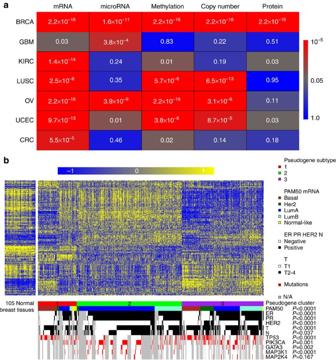Figure 4: Correlations of pseudogene expression subtypes with other tumour subtypes. (a) Concordance between pseudogene expression subtypes and molecular subtypes defined by other genomic data in seven TCGA cancer types. Pseudogene expression subtypes were defined based on the expression of 500 pseudogenes with the most variable patterns through unsupervised analysis using NMF29. The colours indicate the statistical significance of theχ2tests for assessing the concordance between the pseudogene expression subtypes and other molecular subtypes. (b) Concordance between pseudogene expression subtypes and other subtypes in BRCA. Pseudogene expression: subtype 1, red (n=144); subtype 2, green (n=390); subtype 3, and purple (n=303). PAM50 subtypes: basal-like (brown), HER2-enriched (dark green), luminal A (blue), luminal B (aquamarine) and normal-like (yellow). The status of ER, PR, HER2 or N is marked in black (positive) and white (negative); T status is marked in black (T2–T4) and white (T1). Mutations of TP53, PIK3CA, GATA3, MAP3K1 and MAP2K4 are marked in red. Correlations were assessed byχ2tests. Figure 4: Correlations of pseudogene expression subtypes with other tumour subtypes. ( a ) Concordance between pseudogene expression subtypes and molecular subtypes defined by other genomic data in seven TCGA cancer types. Pseudogene expression subtypes were defined based on the expression of 500 pseudogenes with the most variable patterns through unsupervised analysis using NMF [29] . The colours indicate the statistical significance of the χ 2 tests for assessing the concordance between the pseudogene expression subtypes and other molecular subtypes. ( b ) Concordance between pseudogene expression subtypes and other subtypes in BRCA. Pseudogene expression: subtype 1, red ( n =144); subtype 2, green ( n =390); subtype 3, and purple ( n =303). PAM50 subtypes: basal-like (brown), HER2-enriched (dark green), luminal A (blue), luminal B (aquamarine) and normal-like (yellow). The status of ER, PR, HER2 or N is marked in black (positive) and white (negative); T status is marked in black (T2–T4) and white (T1). Mutations of TP53, PIK3CA, GATA3, MAP3K1 and MAP2K4 are marked in red. Correlations were assessed by χ 2 tests. Full size image Here, we present breast cancer as an example ( Fig. 4b ). Based on the NMF consensus clustering, 837 BRCA samples can be classified into four distinct subtypes (cophenetic correlation=0.98, Supplementary Fig. 7 ): subtype 1 ( n =144), subtype 2 ( n =390), and subtype 3 ( n =303) ( Fig. 4b , Supplementary Data 2 ). These pseudogene subtypes show high concordance with the well-established PAM50 molecular subtypes [25] and the status of ER/PR/HER2 markers ( χ 2 test, Fig. 4b ). Subtype 1 is significantly enriched for basal-like samples, containing 70 of 139 basal-like samples; subtype 2 is enriched for luminal A and luminal B samples that 382 of 390 samples are these two subtypes; subtype 3 is enriched for Her2 samples, containing 50 of 67 HER2 samples. The pseudogene expression subtypes also correlate with the mutation status of key cancer genes 13 : subtype 1 shows a depletion of GATA3 mutations; subtype 2 has many samples with PIK3CA mutations; subtype 3 shows a significant enrichment of TP53 mutations. These results strongly indicate that pseudogene expression represents a novel and relevant dimension for investigating cancer-related molecular mechanisms; and integrating it with other molecular data-related analysis may help characterize the molecular basis of tumorigenesis in a more comprehensive way. Prognostic power of pseudogene expression in kidney cancer To study the potential clinical value of pseudogene expression, we examined whether the pseudogene subtypes correlate with clinical outcomes in KIRC. Currently, neither prognostic nor predictive markers are recommended for clinical use by the College of American Pathologists. Based on the 500 pseudogenes with the most variable expression, we were able to classify 446 KIRC samples into two distinct subtypes ( Fig. 5a , Supplementary Data 3 ). Tumour samples in subtype 1 convey a much better patient prognosis ( n =234, survival time of 75.8±3.7 months) than those in subtype 2 ( n =212, survival time of 63.1±3.7 months) ( Fig. 5b , log-rank test P =0.019). To assess whether individual pseudogenes can confer prognostic power given clinical variables, for each pseudogene, we built the full multivariate Cox model, consisting of both clinical variables and the pseudogene expression. We observed an enrichment of pseudogenes (115 out of 500) with a statistically significant P -value (false discovery rate (FDR)<0.05) ( Fig. 5c , Supplementary Data 4 ). Noteworthy, among the 115 pseudogenes, only 19 (16.5%) showed relatively high-expression correlations (Spearman correlation ≥0.5) with their WT genes, suggesting that the predictive power of pseudogene expression is largely independent of the corresponding WT genes. 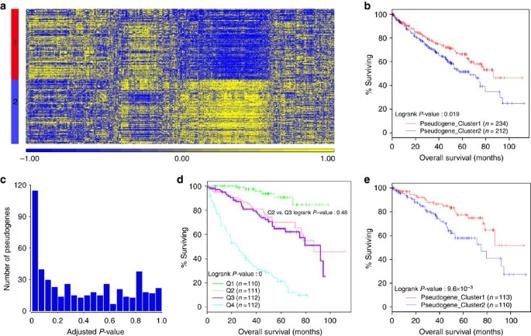Figure 5: Prognostic value of pseudogene expression in KIRC. (a) KIRC subtypes are classified based on the expression of 500 pseudogenes with the most variable patterns through unsupervised analysis using NMF,n=446. (b) Kaplan–Meier plot showing correlations of the two pseudogene expression subtypes with overall survival (log-rank testP=0.019). Red denotes pseudogene expression subtype 1 (n=234); blue denotes pseudogene expression subtype 2 (n=212). (c)P-value distribution of individual pseudogene expressions in multivariate Cox proportional hazards model containing clinical variables. (d) Kaplan–Meier plot of the four risk groups defined by clinical variables in terms of overall survival, and the two middle-risk groups cannot be separated (Q2 (n=111) vs Q3 (n=112), log-rank testP=0.48). (e) Kaplan–Meier plot showing that the two pseudogene expression subtypes can effectively separate the samples in the two medium-risk groups in terms of overall survival (Q2 (n=113) vs Q3 (n=110), log-rank testP=9.6 × 10−3). Figure 5: Prognostic value of pseudogene expression in KIRC. ( a ) KIRC subtypes are classified based on the expression of 500 pseudogenes with the most variable patterns through unsupervised analysis using NMF, n =446. ( b ) Kaplan–Meier plot showing correlations of the two pseudogene expression subtypes with overall survival (log-rank test P =0.019). Red denotes pseudogene expression subtype 1 ( n =234); blue denotes pseudogene expression subtype 2 ( n =212). ( c ) P -value distribution of individual pseudogene expressions in multivariate Cox proportional hazards model containing clinical variables. ( d ) Kaplan–Meier plot of the four risk groups defined by clinical variables in terms of overall survival, and the two middle-risk groups cannot be separated (Q2 ( n =111) vs Q3 ( n =112), log-rank test P =0.48). ( e ) Kaplan–Meier plot showing that the two pseudogene expression subtypes can effectively separate the samples in the two medium-risk groups in terms of overall survival (Q2 ( n =113) vs Q3 ( n =110), log-rank test P =9.6 × 10 −3 ). Full size image To further assess the clinical utility of the observed pseudogene expression subtypes, we classified the KIRC samples into four risk quartiles based on the risk scores (in terms of overall survival) calculated from the multivariate Cox model, employing only clinical variables: low-risk group (Q1, n =110), low-medium-risk group (Q2, n =111), medium-high-risk group (Q3, n =112) and high-risk group (Q4, n =112) (Methods, Supplementary Data 3 ). Although the survival curves of these four risk groups are significantly separated ( Fig. 5d , log-rank test P =0), the clinical variables actually fail to separate the two medium-risk groups ( Fig. 5d , Q2 vs Q3, log-rank test P =0.48). In contrast, the samples in these two groups can be well separated based on the pseudogene expression subtypes ( Fig. 5e , log-rank test P =9.6 × 10 −3 ). For comparison, we performed the same analysis on the two medium-risk groups (Q2 and Q3) using the subtypes defined by mRNA and microRNA expression (obtained from TCGA KIRC Analysis Working Group [15] ) or other molecular data (obtained from TCGA Pan-Cancer Analysis Working Group) and observed no significant correlations with overall survival (log-rank test, mRNA expression, P =0.84; microRNA expression, P =0.13; DNA methylation, P =0.44; somatic copy number alteration, P =0.77; and protein expression, P =0.14). The results in the above survival data analyses underscore the potential prognostic value of pseudogene expression in KIRC. Although they do not generate functional protein products, pseudogenes may act as regulatory RNAs and affect the expression of coding genes through multiple mechanisms [5] . To gain some mechanistic insight into how expressed pseudogenes contribute to the observed KIRC pseudogene expression subtypes, we performed a systematic analysis ( Supplementary Fig. 8a and Supplementary Data 5 ). Among 102 expressed pseudogenes without a clear WT cognate gene, 44 pseudogenes showed a significant differential expression between the two subtypes ( t -test, corrected P <0.05, fold change >1.5), with potential function as lncRNAs [5] . For those pseudogenes with a WT cognate gene, 93 pairs of pseudogenes and their WT genes showed a significant differential expression between the two subtypes ( t -test, corrected P <0.05). Among them, 64 showed strong positive correlations ( R s ≥0.3), suggesting that they may regulate their WT counterparts through competing for shared regulatory RNAs [5] , [30] ; while 4 showed strong negative correlations with their WT cognate genes ( R s ≤−0.3), suggesting that they may function as antisense transcripts to inhibit the WT gene expression. Further analyses on independent, strand-specific RNA-seq data would provide more insights into these mechanisms. Among the WT cognate genes with strong positive correlations with their pseudogenes, we noticed that the survival correlations of individual WT genes with prognostic value match the survival pattern of the pseudogene-expression subtypes: WT genes with better prognosis (potentially tumor suppressors, hazard ratio <1) show higher expression levels in subtype 1 (the better survival group) and the genes with worse prognosis (potentially oncogenes, hazard ratio >1) show higher expression levels in subtype 2 (the worse survival group, Supplementary Fig. 8b ). Finally, we examined the classic miRNA decoy model as proposed in Poliseno et al . (2010) [9] and identified 38 such candidates ( Methods and Supplementary Data 5 ). One candidate of interest is the potential regulation of a putative tumor suppressor a-catenin (CTNNA1) by the pseudogene PGOHUM00000257111 through competition for up to 9 shared miRNA regulators ( Supplementary Data 5 ). Indeed, the expression levels of PGOHUM00000257111 were significantly higher in cluster 1 ( t -test P =1.48 × 10 −7 ), which may lead to the elevated levels of CTNNA1 in subtype 1 ( Supplementary Fig. 8b ) and therefore better survival. Further experimental investigations (for example, cell proliferation assays, siRNA-mediated pseudogene knockdown [10] ) are needed to study these cases in detail. Recently, pseudogenes have emerged as new players in tumour biology [5] , [10] . However, a crucial question remains unclear: does pseudogene expression, as a whole, represent a biologically meaningful dimension that can characterize tumour heterogeneity and provide clinical applications? Here, we performed a Pan-Cancer analysis of pseudogene expression for what is, to our knowledge, the largest number of cancer patient samples (~\n3,000) in one such analysis. Utilizing TCGA patient cohorts with a sufficient sample size, we show the predictive power of pseudogene expression in classifying established tumour types and the high concordance of tumour subtypes based on pseudogene expression with other molecular subtypes as well as clinically established biomarkers (such as ER and PR status in breast cancer). It should be emphasized that a large number of tumour lineage-specific pseudogenes identified through between-disease comparisons [10] do not imply our findings through the within-disease analyses. Because many tumour lineage- or cancer-specific pseudogenes could arise from tissue-related rather than tumorigenesis-related effects, they may or may not have the power to differentiate tumour subtypes. Strikingly, our analysis reveals an unexpected prognostic power of pseudogene expression in kidney cancer: pseudogene expression subtypes not only correlate with patient survival but also confer additional prognostic powers for a group of patients whose survival times cannot be well predicted based on conventional clinical variables. This finding implies a novel prognostic strategy that incorporates both the risk scores defined by the clinical-variable model and the tumour subtypes revealed by pseudogene expression (subtype 1 and subtype 2): among medium-risk patients, patients of subtype 2 may benefit from earlier, more aggressive therapies. Interestingly, although the tumour subtypes defined by other molecular data (for example, mRNA and miRNA) show high concordance with the pseudogene expression subtypes based on the whole patient cohort, they do not confer additional prognostic power based on the medium-risk patient subset. These aggregate results provide a strong rationale for further investigation of the clinical utility of pseudogene expression, which has been understudied in the field. Since TCGA patient samples were collected for the purpose of comprehensive molecular profiling and were collected from different institutions, this practice might introduce some bias. In addition, the resulting clinical annotation of patient samples and related records may not be as rigorous and complete as those obtained from standard clinical trials. Therefore, further efforts should be made to validate the clinical utility of pseudogene expression in a more formal clinical setting (for example, clinical trials). Although our study primarily focused on the biomedical significance and clinical relevance of pseudogene expression as a whole (that is, the subtypes that collectively represent the information of many pseudogenes), an intriguing question is how individual pseudogenes are functionally involved in tumorigenesis. This is a challenging but exciting topic since pseudogenes may affect their WT-coding genes or unrelated genes through multiple mechanisms such as microRNA decoys and antisense transcripts. From a systems biology point of view, the informative behaviour of pseudogenes may originate from a role such as ‘regulator.’ Our preliminary analysis here revealed some candidates of potential interest. Further efforts are required to elucidate how these pseudogenes functionally contribute to tumour initiation and development and how they are regulated through the complex gene regulatory network. Pseudogene expression quantification We downloaded RNA-seq BAM files of 2,808 samples (only primary tumour samples) in seven TCGA cancer types and their related normal tissue samples (if available) from UCSC Cancer Genomics Hub on January, 2013 (CGHub, https://cghub.ucsc.edu/ ). TCGA BAM files were generated based on Mapsplice2 algorithm [32] for alignment against the hg19 reference genome using default parameters. We further filtered the reads mapped with multiple locations in BAM files. To perform a comprehensive survey of pseudogenes, we obtained the genomic information of 16,892 human pseudogenes through combining the latest pseudogene annotations from the Yale Pseudogene Database (build 73) [11] and the GENCODE Pseudogene Resource (version 18) [2] . We further filtered those pseudogene exons that overlapped with any known coding genes. To address the potential cross-mapping issue, we calculated the alignability score [12] for each pseudogene exon. Alignability provides a measure of how often the sequence at a given location will align within the whole genome (up to two mismatches). For each 75-mer window, an alignability score S was defined as 1/(number of matches found in the genome): S =1 means one match in the genome, S =0.5 for two matches in the genome and so on [12] . To count mapped reads for a pseudogene, we only retained those exons with an average alignability score S ≥0.95 to ensure mapping accuracy; and quantified pseudogene expression as RPKM [20] . The pseudogenes with detectable expression were defined as those with an average RPKM ≥0.3 across all samples in each cancer type, as used in the literature [21] , [22] . We then log-transformed the RPKM values for further analysis. We used Spearman rank correlations to assess the co-expression patterns between pseudogenes and their WT cognate genes. The pseudogene expression data have been deposited into Synapse ( https://www.synapse.org/ ) with ID syn1732077. Supervised analysis of expressed pseudogenes To identify tumour lineage-specific/cancer-specific pseudogenes, or those differentially expressed among established molecular or histological subtypes, we used analysis of variance or Student’s t -test to detect the statistical difference between two or more groups. To correct for multiple comparisons, we used the Bonferroni method, with a corrected P -value cutoff of 0.05. To assess the predictive power of pseudogene expression for two UCEC histological subtypes (endometrioid vs serous), we divided the samples into training and test sets according to the institutions where the samples were collected. Adapted from Yuan et al. [33] , we applied three well-established machine-learning algorithms ((RF) [27] , (SVM) [28] and (LR)) to predict the subtype (as a binary variable) using the log-transformed expression levels of pseudogenes (or mRNA) as candidate features. We evaluated the performance of classifiers through fivefold cross-validation within the training set. In detail, we randomly divided the training set into five equal portions; then, during each of the five iterations, we first applied the least absolute shrinkage and selector operator [34] as the feature selection method on 4/5 of the training data and trained the classifiers (1,000 trees for RF, radial kernel for SVM, other parameters set by default) with the selected features. Next, we applied the trained classifiers to the remaining 1/5 of the training data for prediction. The predictions from all five iterations were then combined and compared with the truth, based on which a receiver operating characertistic curve was drawn [35] and the AUC score was calculated accordingly. Finally, we performed feature selection ( Supplementary Data 6 ) and built the classifier from the whole training set using the best-performing algorithm (with the highest AUC) identified through the cross-validation, and applied it to the test set in order to independently validate the predictive power. Analysis of tumour subtypes revealed by pseudogene expression To classify tumour subtypes based on pseudogene expression, for each cancer type, we selected the pseudogenes with the most variable expression pattern (500 for each cancer in the paired-end group and 100 for each cancer in the single-end group), used NMF to classify the tumour samples into clusters [29] and then used the cophenetic correlation to select the optimized clusters. To perform an objective assessment, we obtained independently defined molecular subtypes by other genomic data from TCGA marker papers [13] , [14] , [15] , [16] , [17] , [18] , [19] whenever possible; and if not, then from TCGA Pan-Cancer Analysis Working Group (through a similar NMF-based unsupervised analysis) (syn1688309 for microRNA expression, syn1701558 for DNA methylation and syn1682511 for mRNA expression, copy number variation and protein expression (reverse phase protein array) [36] ). All related subtype classifications and method details are publically available at Synapse [37] . To assess correlations among the subtypes, we used the χ 2 test or Fisher’s exact test, as applicable, and considered P <0.05 to be statistically significant. KIRC patient survival analysis We obtained the clinical information associated with the KIRC samples, including the patient’s overall survival time, age and the tumour grade and stage from TCGA data portal ( https://tcga-data.nci.nih.gov/tcga/ ). We used a log-rank test to examine whether the subtypes significantly correlated with patient survival, and a multivariate Cox proportional hazards model to assess whether the subtype provided additional prognostic power, given the clinical variables; to correct for multiple comparisons, we used the Benjamini–Hochberg method [38] , with an adjusted FDR cutoff of 0.05. To calculate the risk score for patients, we first built a Cox proportional hazard model by fitting the clinical variables (that is, patient age, cancer stage and grade) with the censored survival data, and then plugged the original clinical variables back into the obtained model (that is, the regression function) to calculate the linear predictor or the risk score for each patient. Patients were classified into quartiles grouped by the risk scores (which are essentially continuous values). To display the difference between groups, we used Kaplan–Meier plots, presenting the average survival time as the means±s.e.m., for which we estimated the mean survival time as the area under the survival curve [39] . Mechanistic analysis of pseudogene-driven regulation We downloaded KIRC mRNA expression and miRNA expression from Synapse (syn300013), and used analysis of variance (Bonferroni corrected P <0.05) to identify differentially expressed pseudogenes or mRNAs among the subtypes. We used Spearman rank correlations to assess the expression patterns between a pseudogene and its WT cognate genes: R s ≥0.3 (or ≤−0.3) were considered as strong positive (or negative) correlation. To identify candidates for the miRNA decoy model, we obtained the predicted conserved target sites from MicroRNA.org [40] and used the following criteria: (i) the expression levels of a pseudogene and its WT cognate genes were strongly positively correlated ( Rs ≥0.3); (ii) its WT cognate gene showed a significant negative correlation with the miRNA of interest (FDR<0.05) and contained predicted target sites in its 3′ untranslated region; and (iii) the pseudogene showed a significant negative correlation with the expression of the same miRNA (FDR<0.05). How to cite this article: Han, L. et al. The Pan-Cancer Analysis of pseudogene expression reveals biologically and clinically relevant tumour subtypes. Nat. Commun. 5:3963 doi: 10.1038/ncomms4963 (2014).